Semiconductor-based DNA sequencing of histone modification states The recent development of a semiconductor-based, non-optical DNA sequencing technology promises scalable, low-cost and rapid sequence data production. The technology has previously been applied mainly to genomic sequencing and targeted re-sequencing. Here we demonstrate the utility of Ion Torrent semiconductor-based sequencing for sensitive, efficient and rapid chromatin immunoprecipitation followed by sequencing (ChIP-seq) through the application of sample preparation methods that are optimized for ChIP-seq on the Ion Torrent platform. We leverage this method for epigenetic profiling of tumour tissues. The semiconductor-based, non-optical sequencing technology used by the Ion Torrent sequencer (Life Technologies, Carlsbad, CA) has the potential for scalable, rapid and low-cost sequence data production [1] . Given the current industry standard for the density of transistors on the surface of a semiconductor, the technology has not yet reached its full possible capacity [2] and has the potential to provide comparable sequencing data yields to conventional optical-based sequencers in a fraction of the time and cost [3] , [4] . The technology has recently been applied to genomic sequencing [1] , microbial genotyping [5] and targeted re-sequencing [6] . Chromatin immunoprecipitation followed by high-throughput sequencing (ChIP-seq) is a powerful tool for characterizing the epigenetic landscape and transcriptional network in the context of both normal physiology and disease [7] , [8] , [9] . However, Ion Torrent sequencing has not yet been used for ChIP-Seq because of challenges in using ChIP DNA samples for sequencing library preparation. First, ChIP yields relatively low amounts of DNA, whereas commercial ChIP-Seq protocols recommend at least 500 ng to 1 μg of starting material for the library construction process. This is an issue in particular for ChIP DNA samples from immunoprecipitation of transcription factors or from limiting samples such as rare cell types or clinical samples, which are often at the few nanograms range. Although recent studies presented ChIP-Seq protocols with low input (low cell number) for the Illumina platform [10] , [11] , such protocols are not yet available for the Ion Torrent platform. Second, the Ion Torrent process works optimally with a tight size range of DNA molecules of ~280±20 bp, whereas ChIP DNA typically spans a range of sizes from 200 to 600 bp. Here we demonstrate the utility of Ion Torrent sequencing for ChIP-seq samples with sub-nanogram amounts of DNA. Further, we apply the method to profile epigenetic marks of tumour tissues from melanoma patients and show its potential for analyzing tumour progression. Development of a ChIP-seq application for Ion Torrent Our starting point was an automated 454-library construction method we previously developed [12] . To overcome the low-input material obtained by ChIP, we devised a low input, scalable and robust library construction protocol for ChIP DNA that increases sensitivity and minimizes operator-dependent variability by incorporating a high yielding amplification enzyme (Kapa Biosystems, Woburn, MA), which has higher yield and higher genome coverage [13] than the Phusion polymerase that is commonly used in the standard Illumina protocol, low microlitre volume reactions, molecularly barcoded oligonucleotide adaptors and automated fluid-handling protocols ( Supplementary Fig. S1 and Methods). To address the wide size range of ChIP DNA, we first tested a standard enzymatic DNA-shearing method that is routinely used with Ion Torrent genomic libraries, but failed to generate usable ChIP-Seq libraries. To overcome this problem, we started the library construction process without shearing and then used an automated gel size-selection system (Pippin Prep, Sage Science, Beverly, MA) to select appropriately sized library molecules after adaptor ligation. We note that Illumina ChIP-seq libraries are usually not sheared, as the sheering step results in significant material loss, which is of particular concern with very low-input samples, such as ChIP samples. Using this process, we successfully created libraries for 32 of 36 samples attempted (88.9% pass rate; success defined as having sufficient library material to attempt at least three sequencing reactions. An Illumina ChIP-Seq library construction following a successful ChIP is closer to 100%). To compare results between Ion Torrent sequencing and those from Illumina sequencing for ChIP applications, we performed ChIP with antibodies to the common histone mark, histone 3 lysine 4 tri-methyl (H3K4me3), the carboxy-terminal domain of RNA polymerase II (Pol-II) and IgG (negative control) in mouse dendritic cells stimulated with lipopolysaccharide. The resulting immunoprecipitated DNA was used as an input for both our Ion Torrent and standard Illumina library construction procedures. We sequenced the libraries on the Ion Torrent 316 sequencing chips (on average, two million reads per library, average read length: 180 bases) and with the gold standard ChIP-Seq data production using the Illumina HiSeq 2000 (15 million reads per library; read length: 40 base single end) [7] , [14] , [15] . Illumina has a lower percentage of unmapped bases and a significantly higher rate of well-mapped bases than Ion Torrent ( Supplementary Table S1 ). Although the Ion Torrent reads had higher error rates for both SNPs (10-fold higher) and indels (100-fold higher), these were still below 1 in 1,000 bases ( Supplementary Table S1 ) and thus do not have an impact on the quality of the chromatin maps. We found excellent agreement between the two resulting maps. The ChIP-Seq enrichment scores, defined as the ratio of observed/expected number of reads at each peak region, are highly correlated between the two samples (H3K4me3: Pearson’s R =0.893, Pol-II: R =0.722, Fig. 1a,b ). Despite the differences in mapped bases and error rates, Ion Torrent sequencing produced comparable enrichment peaks to Illumina [5] , [9] , [10] sequencing for both H3K4me3 and Pol-II ChIP-seq ( Fig. 1a,b and Supplementary Fig. S2 ). Saturation analysis by subsampling the Ion Torrent reads indicates that the Ion Torrent library was sequenced to sufficient depth at two million reads ( Fig. 1c ). To examine the possibility that the longer read length in Ion Torrent sequencing reads contributes to this phenomenon, we extended the 40 base reads from Illumina to 180 bases. The extended Illumina reads (randomly down sampled from 15 million to 2 million reads) produced enrichment peaks that were more comparable to the two million Ion Torrent reads, indicating that longer read lengths may be beneficial in ChIP-seq applications independent of the sequencing platform used ( Supplementary Fig. S3 ). Similarly, when we shortened the Ion Torrent reads from 180 bases to 40 bases and then performed alignment, the enrichment peaks were reduced, similar to Illumina reads down sampled to two million reads (40 bases; Supplementary Fig. S3 ). As expected, we did not find enriched peaks with a negative control IgG ChIP-seq from Ion Torrent sequencing ( Supplementary Fig. S4 ). 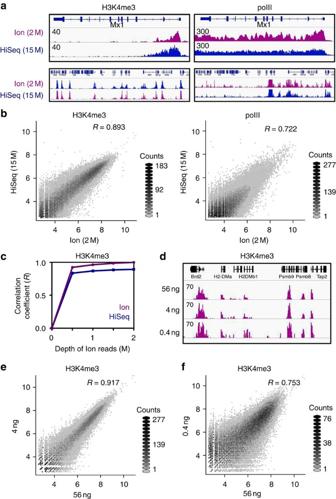Figure 1: Ion Torrent and Illumina HiSeq ChIP-seq. (a) Density profiles of H3K4me3 (left) and Pol-II ChIP-seq (right) from 2 million Ion Torrent reads (purple) and 15 million Illumina HiSeq reads (blue) over theMx1gene locus (top) and a larger region spanning theTNFlocus (bottom). The scale of the density profile was set to the same level for each pair of samples and is marked. All ChIP-seq experiments were performed with mouse dendritic cells stimulated with lipopolysaccharide (0.1 μg ml−1) for 2 h. (b) A comparison of H3K4me3 (left) and Pol-II (right) ChIP-seq peak enrichment scores (log2) over a 500-bp sliding window from 2 million Ion Torrent reads (xaxis) and 15 million Illumina HiSeq reads (yaxis). The Pearson correlation coefficient is marked at the upper right corner. The grey scale represents a two-dimensional density plot, where the grid is divided into hexagonal bins and the colour intensity reflects the density (counts) in the bin. An intensity bar of the counts is shown at the right bottom corner. (c) Saturation analysis to test for sufficient sequencing depth. Shown is the Pearson correlation coefficient (yaxis) calculated between decreasing sequencing reads randomly subsampled from the H3K4me3 ChIP-seq Ion Torrent reads (xaxis) and either 15 million H3K4me3 ChIP-seq Illumina HiSeq reads (blue) or 2 million Ion Torrent reads (purple). (d) Density profiles of H3K4me3 ChIP-seq from 2 million Ion Torrent reads for libraries with 56, 4 or 0.4 ng of immunoprecipitated input DNA. (e,f) A comparison of H3K4me3 ChIP-seq peak enrichment scores (log2) over a 500-bp window from 2 million Ion Torrent reads with 56 ng (yaxis) and 4 ng (d,xaxis) or 0.4 ng (e,xaxis) of immunoprecipitated input DNA. The Pearson correlation coefficient is marked at the upper right corner. The grey scale representation as in panelb. Figure 1: Ion Torrent and Illumina HiSeq ChIP-seq. ( a ) Density profiles of H3K4me3 (left) and Pol-II ChIP-seq (right) from 2 million Ion Torrent reads (purple) and 15 million Illumina HiSeq reads (blue) over the Mx1 gene locus (top) and a larger region spanning the TNF locus (bottom). The scale of the density profile was set to the same level for each pair of samples and is marked. All ChIP-seq experiments were performed with mouse dendritic cells stimulated with lipopolysaccharide (0.1 μg ml −1 ) for 2 h. ( b ) A comparison of H3K4me3 (left) and Pol-II (right) ChIP-seq peak enrichment scores (log 2 ) over a 500-bp sliding window from 2 million Ion Torrent reads ( x axis) and 15 million Illumina HiSeq reads ( y axis). The Pearson correlation coefficient is marked at the upper right corner. The grey scale represents a two-dimensional density plot, where the grid is divided into hexagonal bins and the colour intensity reflects the density (counts) in the bin. An intensity bar of the counts is shown at the right bottom corner. ( c ) Saturation analysis to test for sufficient sequencing depth. Shown is the Pearson correlation coefficient ( y axis) calculated between decreasing sequencing reads randomly subsampled from the H3K4me3 ChIP-seq Ion Torrent reads ( x axis) and either 15 million H3K4me3 ChIP-seq Illumina HiSeq reads (blue) or 2 million Ion Torrent reads (purple). ( d ) Density profiles of H3K4me3 ChIP-seq from 2 million Ion Torrent reads for libraries with 56, 4 or 0.4 ng of immunoprecipitated input DNA. ( e , f ) A comparison of H3K4me3 ChIP-seq peak enrichment scores (log 2 ) over a 500-bp window from 2 million Ion Torrent reads with 56 ng ( y axis) and 4 ng ( d , x axis) or 0.4 ng ( e , x axis) of immunoprecipitated input DNA. The Pearson correlation coefficient is marked at the upper right corner. The grey scale representation as in panel b . Full size image To determine the sensitivity of Ion Torrent sequencing for ChIP-seq, we tested a titration of ChIP DNA input amounts. We used 56, 4 and 0.4 ng of H3K4me3 ChIP DNA from a single ChIP experiment as input for our modified library construction protocol for Ion Torrent. We obtained successful libraries from all three aliquots with comparable results ( Fig. 1d–f ). For example, the lowest input library (0.4 ng; equivalent to H3K4me3-immunoprecipitated DNA from 20,000 cells) was comparable to the highest input library (56 ng; equivalent to 10 × 10 6 cells) based on enriched peaks ( Fig. 1c ) and correlation in enriched scores ( R =0.753, Fig. 1f ). Such low ChIP DNA input amounts are an order of magnitude lower than the Ion Torrent guidelines for library production and sequencing, and are comparable to recently developed protocols [10] , [11] for low input ChIP-seq with the Illumina platform. We also tested 0.05 ng of ChIP DNA, but failed to produce a high-quality library. In summary, using our protocol we created successful libraries from very low starting amounts of ChIP DNA and obtained comparable results with Ion Torrent ChIP-seq to those with our standard methods, optical-based Illumina sequencing, while requiring an order of magnitude fewer sequencing reads (albeit longer reads). Epigenetic signatures during cancer progression The rapid nature and relatively low cost of Ion Torrent sequencing make it a promising candidate for diagnostic applications. As a proof of principal, we next performed H3K4me3 ChIP-seq experiments with a matched pair of primary tumour and metastasis cell lines derived from the same melanoma patient. Although the matched pair WM115 (primary tumour) and WM266-4 (metastasis) showed global correlated enrichment of H3K4me3 in gene promoters ( r 2 R =0.83, Fig. 2a and Supplementary Fig. S5 ), a large number of the genes demonstrated increased levels of H3K4me3 on their promoters in either the primary tumour ( Fig. 2a,b ) or metastasis ( Fig. 2a,c ). To test whether any biological functions were associated with differential levels of H3K4me3, we performed gene set enrichment analysis (GSEA) with the gene sets in the Molecular Signatures Database (MSigDB) [16] . 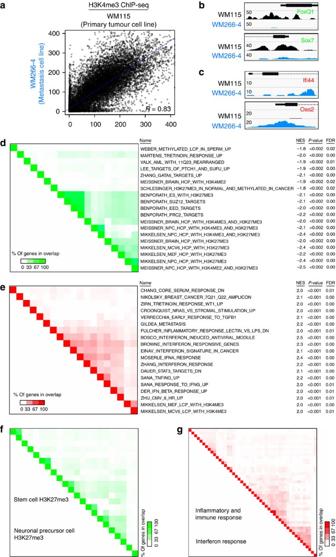Figure 2: Epigenetic signatures correspond to cancer progression. (a) A comparison of accumulated H3K4me3 profiles in a pair of matching metastasis and primary tumour cell lines. Shown are the number of ChIP-seq reads over 1 kb upstream and 1 kb downstream of transcription start site of each of 20,000 human genes in a matched pair of primary melanoma tumour (WM115, black,xaxis) and metastasis (WM266-4, blue,yaxis) cell lines derived from the same patient. The Pearson correlation coefficient is in the bottom right corner. (b,c) Density profiles of normalized reads from H3K4me3 ChIP-seq of primary melanoma tumour-derived cell line (WM115) or metastasis-derived cell line (WM266-4) at illustrative loci with either lower (b) or higher (c) levels of H3K4me3 in the metastasis-derived cell line. (d–g) Gene sets enriched (by GSEA) among loci with different levels of histone modifications. In each case, shown are the names of the enriched gene sets (rows) along with the normalized enrichment score, enrichmentP-value and false discovery rates. Each entry in the heat map indicates the percent overlap in ‘leading edge genes’ (those that contribute to the enrichment) between two enriched gene sets. (d) Genes with lower H3K4me3 in metastasis cell line (WM266-4) relative to control primary tumour cell line (WM115). (e) Genes with higher H3K4me3 in metastasis cell line (WM266-4) relative to control primary tumour (WM115). (f) Genes with lower H3K4me3 in metastatic melanoma tumours from patients (an average of seven tumours samples) relative to control normal skin melanocytes (an average of three biological samples). (g) Genes with higher H3K4me3 in metastatic melanoma tumours from patients relative to control normal skin melanocytes. Figure 2: Epigenetic signatures correspond to cancer progression. ( a ) A comparison of accumulated H3K4me3 profiles in a pair of matching metastasis and primary tumour cell lines. Shown are the number of ChIP-seq reads over 1 kb upstream and 1 kb downstream of transcription start site of each of 20,000 human genes in a matched pair of primary melanoma tumour (WM115, black, x axis) and metastasis (WM266-4, blue, y axis) cell lines derived from the same patient. The Pearson correlation coefficient is in the bottom right corner. ( b , c ) Density profiles of normalized reads from H3K4me3 ChIP-seq of primary melanoma tumour-derived cell line (WM115) or metastasis-derived cell line (WM266-4) at illustrative loci with either lower ( b ) or higher ( c ) levels of H3K4me3 in the metastasis-derived cell line. ( d – g ) Gene sets enriched (by GSEA) among loci with different levels of histone modifications. In each case, shown are the names of the enriched gene sets (rows) along with the normalized enrichment score, enrichment P -value and false discovery rates. Each entry in the heat map indicates the percent overlap in ‘leading edge genes’ (those that contribute to the enrichment) between two enriched gene sets. ( d ) Genes with lower H3K4me3 in metastasis cell line (WM266-4) relative to control primary tumour cell line (WM115). ( e ) Genes with higher H3K4me3 in metastasis cell line (WM266-4) relative to control primary tumour (WM115). ( f ) Genes with lower H3K4me3 in metastatic melanoma tumours from patients (an average of seven tumours samples) relative to control normal skin melanocytes (an average of three biological samples). ( g ) Genes with higher H3K4me3 in metastatic melanoma tumours from patients relative to control normal skin melanocytes. Full size image Interestingly, we found that decreased H3K4me3 levels in metastasis are significantly associated with genes whose expression is repressed in embryonic stem cells, including targets of the polycomb repressive complex and for genes enriched for the H3K27me3 histone mark in embryonic stem cells [17] ( Fig. 2d ). Conversely, increased H3K4me3 levels in metastasis are significantly associated with interferon response and inflammatory response genes ( Fig. 2e ). H3K4me3 is mostly enriched in promoters of actively transcribed genes, whereas H3K27me3 is usually enriched at repressive chromatin regions. In embryonic stem cells, however, many of the polycomb targets, and especially key developmental regulators, are marked by both marks (‘bivalent domains’) [18] . To explore the relationship between these two marks and metastasis, we performed H3K27me3 ChIP-seq experiments in the same cell lines. Indeed, increased H3K27me3 levels in metastasis correlate with loss of H3K4me3 and such genes are enriched for polycomb target genes in embryonic stem cells ( Supplementary Fig. S6a ). Interestingly, genes that have decreased H3K27me3 levels in metastasis are enriched for interferon response genes ( Supplementary Fig. S6b ; a few of the interferon response gene sets are enriched in the top 150 gene sets). To gain initial insight into the clinical applicability of the technology, we performed H3K4me3 ChIP-seq of seven metastatic tumour tissues from melanoma patients. Consistent with our observation in the progressive cell lines, genes that have increased H3K4me3 levels in the metastatic tumours are enriched for interferon, inflammatory and immune response genes and genes that have decreased H3K4me3 levels are enriched for H3K27me3/polycomb target genes ( Fig. 2f,g and Supplementary Figs S7–S10 ). The repression of developmental gene sets in melanoma metastasis by an H3K27me3 gain and H3K4me3 loss is consistent with recent findings of similar embryonic stem cell signatures in aggressive tumours from other cancers [19] , [20] . Further, several reports show that several histone-modifying enzymes are misregulated in human cancers [21] . For example, EZH2, an H3K27me3 writer, is overexpressed in various solid tumours and its expression is correlated with tumour aggressiveness and metastatic progression [22] , [23] . Consistent with this, a stem cell polycomb repression signature is also enriched in genes that gain H3K27me3 marks in metastatic prostate cancer [24] . Our finding that interferon and inflammatory response genes have higher levels of the H3K4me3 mark in melanoma metastasis is consistent with recent findings that link inflammation with cancer [25] , [26] , [27] . In summary, we have demonstrated a rapid, sensitive, scalable and cost-effective semiconductor-based ChIP-seq pipeline for characterizing epigenetic signatures of metastatic human tumours from limiting samples with comparable sensitivity to recently developed protocols [10] , [11] for ChIP-seq with low input using the Illumina platform. The technical and analytical methods for ChIP followed by Ion Torrent sequencing provide a platform for discovery and future diagnostic applications. Cell culture and human tissues Mouse dendritic cells were isolated from wild-type female 6–8-week old C57BL/6 mice obtained from the Jackson Laboratories and cultured in RPMI medium (Invitrogen) supplemented with 10% heat-inactivated fetal bovine serum (Invitrogen) and granulocyte macrophage-colony-stimulating factor (20 ng ml −1 ; Peprotech, Rocky Hill, NJ) [28] . Cells were cultured for 9 days and stimulated for 2 h with lipopolysaccharide (100 ng ml −1 , rough, ultrapure Escherichia coli K12 strain). Paired primary melanoma tumour-derived cell line (WM115) and metastatic melanoma tumour-derived cell line (WM266-4) from the same patient were obtained from the Wistar Institute (Philadelphia, PA). Metastatic melanoma tissues were collected from the Department of Surgical Oncology, University of Texas, MD Anderson Cancer Center with informed consent of the patients and prior MIT Committee On the Use of Humans as Experimental Subjects approval. ChIP assay ChIP assays were performed using a previously published protocol with some minor modifications [28] . Briefly, cells were fixed for 10 min with 1% formaldehyde and quenched with glycine. Cells were lysed for 10 min on ice with RIPA lysis buffer (10 mM Tris–HCl pH 8.0, 1 mM EDTA pH 8.0, 140 mM NaCl, 1% Triton X-100, 0.1% SDS, 0.1%; sodium deoxycholate for mouse dendritic cells) or RIPA lysis buffer with 0.2% SDS and without Triton X-100 (for WM115 and WM266-4 melanoma cell lines) and then sonicated using the Branson sonicator as described in Garber et al . [28] Frozen human melanoma tissues (50–100 mg) were thawed out on ice and chopped finely with a razor blade. Then tissues were fixed for 10 min with 1% formaldehyde in PBS buffer and quenched with glycine. Fixed tissues were pulverized with Covaris CryoPrep CP02 at setting 5 for two times in TT1ET tissue tube. Cells were lysed for 10 min on ice with 1% SDS lysis buffer (1% SDS, 10 mM EDTA, 50 mM Tris-HCl, pH 8.1) and then sonicated using the Branson sonicator. Immunoprecipitation was performed by incubation of the sonicated cell lysate with 75 μl of protein G magnetic dynabeads (Invitrogen) coupled to target antibody for overnight at 4°C. Magnetic beads were then washed five times with cold RIPA buffer (10 mM Tris–HCl, pH 8.0, 1 mM EDTA, pH 8.0, 140 mM NaCl, 1% Triton X-100, 0.1% SDS), twice with high-salt RIPA buffer (10 mM Tris–HCl, pH 8.0, 1 mM EDTA, pH 8.0, 500 mM NaCl, 1% Triton X-100, 0.1% SDS), twice with LiCl buffer (10 mM Tris–HCl, pH 8.0, 1 mM EDTA, pH 8.0, 250 mM LiCl, 0.5% NP-40, 0.5% sodium deoxycholate), twice with TE buffer, and then eluted in 50 μl of elution buffer (10 mM Tris–HCl, pH 8.0, 5 mM EDTA, pH 8.0, 300 mM NaCl and 0.5% SDS). The eluate was reverse crosslinked at 65°C for 6 h and then treated with 2 μl of RNase A (Roche Applied Science) for 30 min and 2.5 μl of proteinase K (Invitrogen) for 2 h. Finally, the de-crosslinked DNA samples were cleaned up with 120 μl of solid-phase reversible immobilization (SPRI) beads and eluted in 50 μl of EB buffer (10 mM Tris–HCl, pH 8.0). Ion Torrent library production and sequencing ChIP-Seq libraries for Ion Torrent sequencing were created using a modified protocol of the manufacturer’s instructions. The process for sample preparation is outlined in Supplementary Fig. S1 . Briefly, 45 μl of each ChIP DNA was added to a 96-well microtiter plate. Physical barcoding of all sample receptacles was employed at each step to ensure sample tracking integrity. Fragments were enzymatically end-repaired using an enzyme and buffer cocktail (Kapa Biosystems). Following end-repair, automated reaction clean-up was performed using a SPRI process with a ratio of 1.8 times beads to DNA (Ampure, Agencourt, Beckman Coulter). Samples were eluted in 30 μl and added to a 50-μl adaptor ligation reaction (ligase enzyme and buffer from Kapa Biosystems), which also contained 5 μl of Ion Torrent compatible oligonucleotide adaptors (Integrated DNA Technologies). Adaptors were used at 8 μM concentration (one-fifth of the standard amount) to minimize adaptor dimer with the low-input samples. A further 1.8 × SPRI was performed after adaptor ligation. All automated fluid-handling steps were carried out on a Bravo Automated Liquid Handling Platform, with a 96LT Disposable Tip pipette head (Agilent Technologies, Santa Clara, CA). After adaptor ligation, 10 μl of loading solution was added to each sample and each sample was size selected (280 base target size) using 2% gel cartridges (SAGE Pippin prep, Sage Science). A further SPRI (2 × Bead:DNA ratio) was performed after sizing and samples were eluted in 23 μl volume. An amplification reaction was set up in a final volume of 50 μl with the following cycling profile: 98 °C for 45 s; 72 °C for 20 min; followed by 12 cycles of 98 °C for 15 s, 63 °C for 30 s and 72 °C for 30 s; and finally, 72 °C for 60 s. Amplification enzymes and master mix were from Kapa Biosystems, and primers were those provided in the Ion Torrent template preparation kit. A SPRI clean-up with a 1.5 × Bead:DNA ratio was performed after amplification and final libraries were eluted in 25 μl volume. Libraries were quantified and checked for size on an Agilent Bioanalyzer (Agilent Technologies). Template preparation was conducted using the Ion PGM 200 Xpress Template Kit, following the Ion PGM 200 Xpress Template Kit protocol (version 3). Libraries were diluted and 18 μl of the 1.55 × 10 7 molecules per μl dilution was added to an aqueous master mix containing polymerase and ion sphere particles (ISPs) according to the manufacturer’s specified proportions. Emulsions were created using an IKA Ultra-Turrax Tube Drive (IKA, Wilmington, NC). After emulsion PCR, DNA-positive ISPs were recovered and enriched according to standard protocols. A sequencing primer was annealed to DNA-positive ISPs and the sequencing polymerase was bound before loading of ISPs into Ion 316 sequencing chips. Sequencing of the samples was conducted according to the Ion PGM 200 Sequencing Kit Protocol (version 6). One or more 316 sequencing chips were loaded and run on an Ion Personal Genome Machine for each sample. Each run was programmed to include 520 nucleotide flows to deliver 200 base read lengths on average. Libraries were sequenced on Ion Torrent Personal Genome Machine. Base calling and alignment were performed by the Torrent Suite 2.0.1 software. Illumina library production and sequencing ChIP-seq library for Illumina sequencing were prepared using a previously published protocol [28] . Briefly, enzymes from New England Biolabs were used for the following library construction processes, DNA end-repair, A-base addition and adaptor ligation, and Pfu Ultra II fusion enzyme (Agilent Technologies) was used for the enrichment step. Illumina ChIP libraries were barcoded and pooled as previously described [28] . ChIP-seq analysis Reads were aligned to the reference mouse genome (mm9) or human genome (hg19) using the BWA aligner version 0.5.9. Sequencing metrics were extracted using the GATK tools [29] to traverse the genome and qualify mapped bases as well aligned—when the reads had mapping quality greater than Q20 (phred scaled) and high quality—when the reads had mapping quality greater than Q20 and the base had base quality greater than Q20. Error rates were measured in every 100 bases. Mismatches were counted for every base that mismatched the reference sequence in the alignment. Insertions and deletions were counted as events (not by the number of bases in the events). The rate is the number of insertion or deletion events found in every 100 bases. Read length was calculated over all reads (including unmapped). Unmapped reads are all the reads that did not find a likely mapping in the mouse reference genome mm9 (this does not include mapping quality 0 reads). ChIP-seq peak calling was performed using the contiguous segmentation algorithm as part of the Scripture package [28] ( http://www.broadinstitute.org/software/scripture/ ). Pearson’s correlation coefficients in Fig. 1 were calculated by performing Pearson’s correlation analysis of pairwise comparison of ChIP-seq peak enrichment scores (log2) over a 500-base sliding window. To simulate for longer reads, we extended the 40-base Illumina reads to 180 bases by setting the extFactor flag to 140 in igvtools ( http://www.broadinstitute.org/software/igv/igvtools_commandline ). To simulate for shorter Ion Torrent reads, we selected the first 40 bases from the 180 bases of Ion Torrent reads. The sequencing data can be downloaded from the NCBI GEO database with the following accession number GSE49477. GSEA analysis GSEA v2.2 was used to test for enrichment of each of the 3,398 gene sets in the chemical and genetic perturbation collection of the Molecular Signature Database (MSigDB v3.1). Reads were first normalized based on the total number of reads for each sample. For each of the 20,000 NCBI human Refseq genes, the accumulated H3K4me3 ChIP-seq reads over 1 kb upstream and 1 kb downstream of transcription start site was calculated to present the H3K4me3 ChIP-seq signal for each gene. The residuals of the natural logarithms of the accumulated reads calculated from the linear model for each gene were used as the ranked list input for the GSEAPreranked function. Three biological repeats of H3K4me3 ChIP-seq Illumina sequencing data from normal skin melanocytes were downloaded from NCBI GEO database (GSE16368) [30] . Accession Codes: Sequencing data have been uploaded to the NCBI GEO database under Accession Number GSE49477 . How to cite this article: Cheng, C. S. et al . Semiconductor-based DNA sequencing of histone modification states. Nat. Commun. 4:2672 doi: 10.1038/ncomms3672 (2013).